The same self-peptide selects conventional and regulatory CD4+T cells with identical antigen receptors The role of the T-cell receptor (TCR) in commitment of thymocytes to regulatory CD4 + Foxp3 + and conventional CD4 + Foxp3 − T-cell lineages remains controversial. According to the prevailing view, commitment to the former lineage, in contrast to the latter, requires that high affinity TCRs bind rare class II MHC/peptide complexes presented in ‘thymic niches’, which could explain differences between their TCR repertoires. Here we challenge this view and show that the binding of identical TCRs to the same ubiquitously expressed MHC/peptide complex often directs thymocytes to both CD4 + lineages, indicating that the TCR affinity does not play the instructive role, and that restricted presentation of peptides in ‘thymic niches’ is not necessary for selection of CD4 + Foxp3 + T cells. However, depending on whether immature thymocytes bound the ligand predominantly with low or high affinity, the repertoires of regulatory and conventional CD4 + T cells were correspondingly similar or mostly different, suggesting that negative rather than positive selection sets them apart. The primary repertoire of αβ T-cell receptors (TCR) is shaped by positive and negative selection of immature CD4 + CD8 + thymocytes whose fate depends on the strength of the TCR signal, triggered by the recognition of self-peptides bound by major histocompatibility complex (MHC) molecules. The TCR affinity for selecting peptide and the number of TCR engaged (that is, avidity) are two essential factors determining the strength of this signal. Thymocytes that receive signals that are too weak or too strong are negatively selected and die by apoptosis, while those that receive signals of intermediate strength are positively selected, survive and differentiate [1] , [2] . Thymocytes positively selected by peptides bound by class II MHC molecules differentiate to two functionally different CD4 + T cells: regulatory (Treg, CD4 + Foxp3 + ) and conventional (CD4 + Foxp3 − ; refs 3 , 4 ). A question that remains unresolved is whether commitment to these T-cell lineages occurs within the same or different range of TCR affinities. Several studies suggested that commitment to CD4 + Foxp3 + , in contrast to CD4 + Foxp3 − lineage, depends on relatively high affinity interactions of TCRs with rare, tissue-specific self-peptides presented in ‘thymic niches’ [5] , [6] , [7] , [8] , [9] , [10] , which could be responsible for the observed differences between their TCR repertoires [11] , [12] , [13] . On the other hand, recent studies showed that the TCR repertoires of these two subsets of CD4 + T cells, as well as the range of TCR affinities supporting their positive selection, are considerably overlapping [14] , [15] . This observation implied that the commitment to CD4 + Foxp3 + and CD4 + Foxp3 − lineages is not guided by the TCR affinity for positively selecting peptide. However, since in all these studies the selecting peptides were not identified, the possibility that CD4 + Foxp3 + and CD4 + Foxp3 − thymocytes expressing the same TCRs were selected by different self-peptides recognized with different affinities, could not be excluded. Alternatively, the differences between the TCR repertoires of conventional and regulatory T cells could be imposed by negative selection because the susceptibility to apoptosis of CD4 + Foxp3 + and CD4 + Foxp3 − thymocytes was shown to be different [16] , [17] , [18] . To address these questions we compared repertoires of CD4 + Foxp3 + and CD4 + Foxp3 − thymocytes selected on class II MHC molecules bound exclusively with one or another variant of self-peptide recognized by predominant fraction of immature thymocytes with low or high affinity, respectively. We show that in both cases the binding of identical TCRs to the same ubiquitously expressed MHC/peptide complex often directs thymocytes to both CD4 + lineages, indicating that the TCR affinity does not play a role in selecting one over the other, and that selection of regulatory CD4 + T cells can occur on peptides with unrestricted thymic expression. However, depending on the bias of the primary TCR repertoire to bind the selecting ligand with low or high affinity, the resulting repertoires of regulatory and conventional CD4 + T cells were correspondingly similar or mostly different, suggesting that negative rather than positive selection is responsible for their separation. Generation of CD4 + T cells in ‘single-peptide’ TCR mini mice To study the impact of TCR affinity on the commitment of thymocytes to CD4 + Foxp3 + and CD4 + Foxp3 − lineages and on their TCR repertoires, we first analyzed the generation of CD4 + T cells in ‘single-peptide’ mice, which express a limited TCR repertoire (TCR mini ; ref. 19 ) and class II MHC molecules (A b ) that are exclusively bound with Eα(52–68) peptide (Ep) or its analogue Ep63K (Ep63K). We crossed these mice to Foxp3 GFP reporter [20] mice, generating TCR mini Foxp3 GFP strain (referred to hereon as TCR mini ). The expression levels of A b Ep and A b Ep63K complexes on thymic epithelial cells are very similar and resemble that of native A b Ep complexes in congenic B10.5R mice [21] , [22] , [23] . Moreover, the timing of TCR expression on immature thymocytes in TCR mini mice resembles the timing in wild-type (A b wt) mice, and CD4 + thymocytes differentiate into CD4 + Foxp3 − or CD4 + Foxp3 + lineages [19] ( Fig. 1a first column, and Fig. 2a ). The TCR genes used to create TCR mini mice were derived from a T cell originally selected by A b Ep complex, which recognized the A b Ep63K complex as cognate antigen [24] . It was therefore expected that in A b Ep63KTCR mini mice a larger proportion of CD4 + CD8 + thymocytes will bind selecting complex with high affinity than in A b EpTCR mini mice, while in A b EpTCR mini mice a larger proportion of CD4 + CD8 + thymocytes will bind selecting complex with low affinity than in A b Ep63KTCR mini mice. Importantly, due to the saturation of all A b molecules with identical peptide, the possible differences in TCR avidity between individual thymocytes expressing identical TCRs were maximally reduced making these mice uniquely suitable to study the role of TCR affinity in commitment to CD4 + Foxp3 + and CD4 + Foxp3 − lineages. 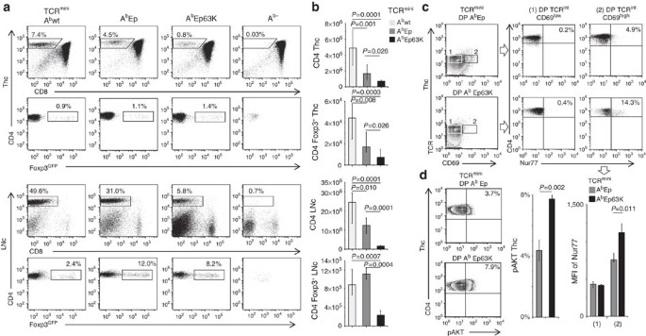Figure 1: Generation and phenotype of CD4+thymocytes and T cells in ‘single-peptide’ TCRminimice. (a) Representative phenotypes of thymocytes (Thc) and lymph node cells (LNc) from indicated strains of mice. Numbers indicate the proportions of CD4+and CD4+Foxp3+cells. (b) Total numbers of CD4+and CD4+Foxp3+cells in the thymus (upper panel) and lymph nodes (lower panel) of indicated mice. Bars show the mean (±s.d.) of two independent experiments, in which at least four mice per group were analyzed. (c). Expression of CD69 and Nur77 on CD4+CD8+(DP) thymocytes. (d). Expression of phosphorylated AKT in DP thymocytes from indicated mice. Bars show the mean (±s.d.), and represent data from three to five mice. Statistical significance of data was calculated using two-samplet-test (OriginLab). GFP, green fluorescent protein. Figure 1a shows that, in contrast to the A b -deficient TCR mini mice, both ‘single-peptide’ TCR mini mice supported the development of a substantial number of CD4 + Foxp3 + and CD4 + Foxp3 − thymocytes, although the proportions and total numbers of thymic and peripheral CD4 + T cells generated in these mice, due to the absence of peptide diversity, were lower than in the A b wtTCR mini mice. Interestingly, the reduction in the A b EpTCR mini mice was much weaker than in the A b Ep63KTCR mini mice ( Fig. 1a,b ), which had higher proportion of CD4 + CD8 + thymocytes with elevated expression of activation markers such as Nur77 and phosphorylated AKT kinase ( Fig. 1c,d ), which are associated with TCR-mediated signalling [25] , [26] . This observation suggested that lower number of CD4 + T cells generated in A b Ep63KTCR mini mice could be the consequence of higher proportion of thymocytes undergoing apoptosis, reflecting higher proportion of thymocytes recognizing the cognate ligand with high affinity. In agreement with this possibility, the proportion of apoptotic cells among CD4 + CD8 + CD69 high CD5 int thymocytes, which undergo selection but not among post-selected CD69 high CD5 high cells [25] , was much higher in A b Ep63KTCR mini than in A b EpTCR mini mice ( Fig. 2b,c ). Interestingly, in spite of the lower numbers of CD4 + T cells, the proportion of CD4 + Foxp3 + to CD4 + Foxp3 − cells in both ‘single-peptide’ mice was higher than in A b wtTCR mini mice ( Fig. 1a ), possibly reflecting higher resistance of CD4 + Foxp3 + thymocytes to TCR-mediated deletion [16] , [17] , [27] . The above results showed that thymus-derived regulatory CD4 + Foxp3 + T cells (tTregs), can be generated in mice expressing only single, ubiquitously expressed A b /peptide complex, and confirmed the initial assumption that in the A b Ep63KTCR mini mice more immature thymocytes recognized cognate ligand with affinities from the high end of the spectrum than in the A b EpTCR mini mice, as indicated by higher proportion of immature thymocytes undergoing apoptosis. Figure 1: Generation and phenotype of CD4 + thymocytes and T cells in ‘single-peptide’ TCR mini mice. ( a ) Representative phenotypes of thymocytes (Thc) and lymph node cells (LNc) from indicated strains of mice. Numbers indicate the proportions of CD4 + and CD4 + Foxp3 + cells. ( b ) Total numbers of CD4 + and CD4 + Foxp3 + cells in the thymus (upper panel) and lymph nodes (lower panel) of indicated mice. Bars show the mean (±s.d.) of two independent experiments, in which at least four mice per group were analyzed. ( c ). Expression of CD69 and Nur77 on CD4 + CD8 + (DP) thymocytes. ( d ). Expression of phosphorylated AKT in DP thymocytes from indicated mice. Bars show the mean (±s.d. ), and represent data from three to five mice. Statistical significance of data was calculated using two-sample t -test (OriginLab). GFP, green fluorescent protein. 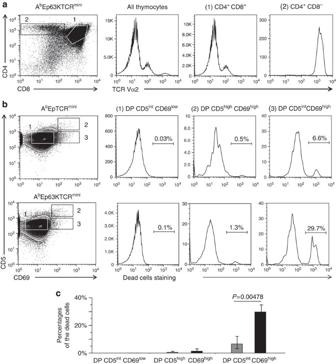Figure 2: Apoptosis of immature Vα2+CD5+CD69+thymocytes in AbEp63KTCRminiand in AbEpTCRminimice. (a) Representative TCR expression pattern on thymocytes (gated as shown) from AbEpTCRminiand AbEp63KTCRminimice (thymocytes from AbEp63KTCRminimice are shown). (b) Staining by the LIVE/DEAD Fixable Far-Red Dead Cell Stain Kit of CD5/CD69 subpopulations of CD4+CD8+(DP) thymocytes from AbEpTCRminior AbEp63KTCRminimice, gated as shown. (c) An average proportion of apoptotic thymocytes in AbEpTCRmini(grey bars) or AbEp63KTCRmini(black bars) mice (±s.d.). Five mice per group were analyzed. One-way analysis of variance was used as statistical method. Full size image Figure 2: Apoptosis of immature Vα2 + CD5 + CD69 + thymocytes in A b Ep63KTCR mini and in A b EpTCR mini mice. ( a ) Representative TCR expression pattern on thymocytes (gated as shown) from A b EpTCR mini and A b Ep63KTCR mini mice (thymocytes from A b Ep63KTCR mini mice are shown). ( b ) Staining by the LIVE/DEAD Fixable Far-Red Dead Cell Stain Kit of CD5/CD69 subpopulations of CD4 + CD8 + (DP) thymocytes from A b EpTCR mini or A b Ep63KTCR mini mice, gated as shown. ( c ) An average proportion of apoptotic thymocytes in A b EpTCR mini (grey bars) or A b Ep63KTCR mini (black bars) mice (±s.d.). Five mice per group were analyzed. One-way analysis of variance was used as statistical method. Full size image The same peptide selects CD4 + Foxp3 + and Foxp3 − cells with identical TCRs Because A b EpTCR mini and A b Ep63KTCR mini mice differ in the extent of intrathymic apoptosis, comparison of TCR repertoires of CD4 + Foxp3 + and CD4 + Foxp3 − thymocytes in these mice could be informative as to the significance of negative selection in shaping their repertoires. We also thought that if TCR affinity plays critical role in the commitment, the TCR repertoires of CD4 + Foxp3 + and CD4 + Foxp3 − thymocytes positively selected on the same, single peptide should be largely non-overlapping. Conversely, if the affinity of TCR-ligand interaction does not dictate the commitment, the repertoires should be largely overlapping. To analyze TCR repertoires we used high-throughput sequencing. Figure 1a and Supplementary Figure 1a show that as in A b -deficient (A b− ) mice with unlimited TCR repertoire [16] , some CD4 + T cells were also found in A b− TCR mini mice. TCRs sequenced from these cells accounted for 20–40% of TCR mini repertoires selected on A b Ep or A b Ep63K complexes ( Fig. 3a,b grey slices). These sequences (their frequencies in different TCR mini strains are shown in Supplementary Fig.1b ) were excluded from further analysis to eliminate TCRs that could be selected on ligands not associated with class II MHC molecules. 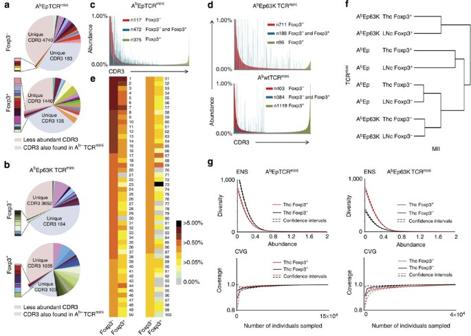Figure 3: CD4+Foxp3+and CD4+Foxp3−thymocytes selected on the same peptide often express identical TCRs. (a,b) Pie charts depict the 20 most dominant TCRα CDR3 regions from CD4+Foxp3+and CD4+Foxp3−thymocytes selected on AbEp or AbEp63K complexes. Each dominant CDR3 is represented by a unique colour, and the size of the slice represents its frequency (for sequences seeSupplementary Fig. 2a,b). Protruding slices indicate the abundant TCRs on CD4+Foxp3−thymocytes, found on CD4+Foxp3+thymocytes at low abundance and vice versa. Pink and grey slices depict, respectively, the portions of the repertoires that cover all less abundant CDR3 regions or CDR3 regions also found on CD4+T cells from Ab−TCRminimice (numbers indicate unique CDR3 sequences) (see alsoSupplementary Fig. 1b). (c,d) Charts show the frequencies of individual TCRs found in CD4+Foxp3−and in CD4+Foxp3+repertoires. TCRs accounting for no less than 0.01% in at least one of these repertoires are shown. The frequencies of TCRs found exclusively in Foxp3−repertoire are depicted by the height of the red lines while the frequencies of TCRs found exclusively in Foxp3+repertoire are depicted by the height of the green lines. The TCRs found in both repertoires are marked by blue line. The height of the blue line indicates the frequency in the Foxp3+repertoire, while the frequency in Foxp3−repertoire is indicated by the slope of the red lines histogram (e). 100 most dominant TCRs expressed on CD4+Foxp3−thymocytes in AbEpTCRminimice. Their frequencies on CD4+Foxp3+thymocytes (confirmed by TCR sequencing from single sorted thymocytes19) are shown asSupplementary Fig. 3(f) The hierarchical clusters depict similarity of TCR repertoires based on comparative analysis of the overlap using mutual information index (MII) (based on high-throughput sequencing, seeSupplementary Table 1for the number of TCR CDR3 sequences analyzed). (g) Diversity indices, that is, effective number of species (ENS) and sample coverage (CVG) of TCRα CDR3 repertoires from CD4+Foxp3+and CD4+Foxp3−thymocytes were calculated as described in Methods. TCR sequences were retrieved from indicated subsets from three mice of each kind, isolated and sequenced separately. Figure 3a,b and Supplementary Figure 2a,b also show that within 20 most abundant TCRs found on each subset of CD4 + thymocytes, several were abundant on both subsets. Most TCRs abundant on CD4 + Foxp3 + thymocytes were found at low abundance on CD4 + Foxp3 − thymocytes and vice versa, suggesting that qualitative differences between the repertoires may be in fact smaller than that revealed by the present limited analysis. The observed differences in the frequencies of shared TCRs in CD4 + Foxp3 + and CD4 + Foxp3 − subsets may result from different proliferation rate, thymic dwell time and stochastic events before and/or after selection. The expression of identical TCRs on CD4 + Foxp3 + and CD4 + Foxp3 − thymocytes was previously observed in wt mice [11] , [19] but their expression on both subsets in ‘single-peptide’ mice excluded the possibility that these TCRs were selected on different self-peptides recognized with different affinities. To compare the repertoires of CD4 + Foxp3 + and CD4 + Foxp3 − thymocytes more comprehensively, we examined the TCRs that accounted for no less than 0.01% in at least one sequenced population. Figure 3c shows the alignment of individual CDR3 regions of TCRα chain from CD4 + Foxp3 − thymocytes of A b EpTCR mini mice according to their frequency, overlaid by CDR3 regions from CD4 + Foxp3 + thymocytes. This analysis revealed (in line with the results obtained by single cell PCR, ref. 19 ) that in A b EpTCR mini mice 50% of examined TCRs—each different TCR was counted as one, irrespective of its frequency—were shared by both subsets of CD4 + thymocytes ( Fig. 3c ), demonstrating that binding to the same MHC/peptide ligand frequently directed thymocytes with identical TCRs to different CD4 + lineages (see also Fig. 3e and Supplementary Fig. 3 ). However, the proportion of TCRs shared between CD4 + Foxp3 + and CD4 + Foxp3 − repertoires was lower in A b Ep63KTCR mini and in A b wtTCR mini mice (20 and 18%, respectively, Fig. 3d ), indicating that in mice, in which negative selection was more extensive, the similarity of TCR repertoires was strongly reduced. This conclusion was supported by the calculated similarity indices [28] , which placed the repertoires of CD4 + Foxp3 + and CD4 + Foxp3 − thymocytes from A b Ep63KTCR mini mice on the most extreme opposite branches of the illustrating dendrogram ( Fig. 3f ), while the corresponding CD4 + lineages from A b EpTCR mini mice clustered in close proximity. To determine whether reduced similarity of TCR repertoires of CD4 + Foxp3 + and CD4 + Foxp3 − thymocytes in A b Ep63KTCR mini mice, as compared with A b EpTCR mini mice, is associated with their reduced diversity, and if so, applies to both subsets or to one of them, we used TCR libraries prepared from the same number of CD4 + Foxp3 + and CD4 + Foxp3 − thymocytes. This analysis revealed that in A b EpTCR mini mice, the diversity of TCR repertoires of CD4 + Foxp3 + and CD4 + Foxp3 − thymocytes was comparable, but in A b Ep63KTCR mini mice the diversity of TCRs on CD4 + Foxp3 − thymocytes was significantly reduced ( Fig. 3g ). This last finding suggested that the dissimilarity between repertoires of CD4 + thymocytes committed to conventional and regulatory lineages in A b Ep63KTCR mini mice is primarily a consequence of enhanced negative selection of CD4 + Foxp3 − thymocytes. Figure 3: CD4 + Foxp3 + and CD4 + Foxp3 − thymocytes selected on the same peptide often express identical TCRs. ( a , b ) Pie charts depict the 20 most dominant TCRα CDR3 regions from CD4 + Foxp3 + and CD4 + Foxp3 − thymocytes selected on A b Ep or A b Ep63K complexes. Each dominant CDR3 is represented by a unique colour, and the size of the slice represents its frequency (for sequences see Supplementary Fig. 2a,b ). Protruding slices indicate the abundant TCRs on CD4 + Foxp3 − thymocytes, found on CD4 + Foxp3 + thymocytes at low abundance and vice versa. Pink and grey slices depict, respectively, the portions of the repertoires that cover all less abundant CDR3 regions or CDR3 regions also found on CD4 + T cells from A b− TCR mini mice (numbers indicate unique CDR3 sequences) (see also Supplementary Fig. 1b ). ( c , d ) Charts show the frequencies of individual TCRs found in CD4 + Foxp3 − and in CD4 + Foxp3 + repertoires. TCRs accounting for no less than 0.01% in at least one of these repertoires are shown. The frequencies of TCRs found exclusively in Foxp3 − repertoire are depicted by the height of the red lines while the frequencies of TCRs found exclusively in Foxp3 + repertoire are depicted by the height of the green lines. The TCRs found in both repertoires are marked by blue line. The height of the blue line indicates the frequency in the Foxp3 + repertoire, while the frequency in Foxp3 − repertoire is indicated by the slope of the red lines histogram ( e ). 100 most dominant TCRs expressed on CD4 + Foxp3 − thymocytes in A b EpTCR mini mice. Their frequencies on CD4 + Foxp3 + thymocytes (confirmed by TCR sequencing from single sorted thymocytes [19] ) are shown as Supplementary Fig. 3 ( f ) The hierarchical clusters depict similarity of TCR repertoires based on comparative analysis of the overlap using mutual information index (MII) (based on high-throughput sequencing, see Supplementary Table 1 for the number of TCR CDR3 sequences analyzed). ( g ) Diversity indices, that is, effective number of species (ENS) and sample coverage (CVG) of TCRα CDR3 repertoires from CD4 + Foxp3 + and CD4 + Foxp3 − thymocytes were calculated as described in Methods. TCR sequences were retrieved from indicated subsets from three mice of each kind, isolated and sequenced separately. Full size image Impact of negative selection on TCR repertoire To further investigate the role of negative versus positive selection in separation of TCR repertoires of CD4 + Foxp3 + and CD4 + Foxp3 − thymocytes we also analyzed A b EpTCR mini →A b Ep63KTCRα − chain-deficient (TCRα − ) and A b Ep63KTCR mini →A b EpTCRα − irradiation chimeras [29] . In the first type of chimera Ep peptide was expressed on bone marrow-derived cells, which primarily mediate negative selection, while Ep63K peptide was expressed on thymic epithelial cells, which primarily mediate positive selection [30] . In the second type of chimera the expression pattern of selecting peptides was reversed. The results are shown in Fig. 4 . Thymii from both types of chimeras had similar proportions of CD4 + Foxp3 + and CD4 + Foxp3 − thymocytes ( Fig. 4a ), but their TCR repertoires resembled those of the donor of bone marrow cells, confirming the dominant role of negative selection in setting these repertoires apart (compare Fig. 4b–d with Fig. 3a–d, f ). Furthermore, in A b EpTCR mini →Ep63KTCRα chimera, positive selection of CD4 + Foxp3 + thymocytes was not significantly enhanced, even though negative selection, due to the absence of this complex on bone marrow-derived cells was reduced. Accordingly, similarity analysis showed ( Fig. 4d ) that repertoires from A b EpTCR mini mice clustered with repertoires from A b Ep63KTCR mini mice reconstituted with A b EpTCR mini bone marrow, and were separate from the rest of the repertoires selected in the presence of A b Ep63K complexes on bone marrow-derived cells. Analysis of the diversity and richness of TCRs in chimeric mice also showed that introduction of A b Ep63K complex to mice expressing exclusively A b Ep complex, reduced this repertoire in size and diversity, particularly in case of the CD4 + Foxp3 − subset ( Fig. 4e ), confirming the dominant impact of negative selection on allocation of particular TCRs to given subset of CD4 + thymocytes. 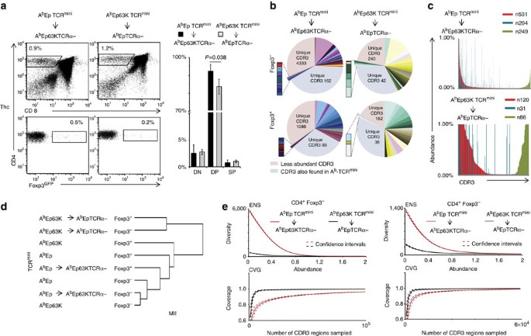Figure 4: Negative selection sets apart TCR repertoires of CD4+Foxp3+and CD4+Foxp3−thymocytes. (a) Phenotype and recovery of thymocytes from the indicated bone marrow chimeras 6 weeks after bone marrow transplantation. Numbers indicate proportions of gated cells, and bar graphs show the mean values ±s.d. from two experiments (four mice per group). Statistical significance of data was calculated using two-samplet-test (OriginLab). (b) Repertoire of TCRαCDR3 regions from CD4+Foxp3−and CD4+Foxp3+thymocytes from indicated chimeras. Colour coding of the particular TCRs is the same as inFig. 3a,b, andSupplementary Fig. 4shows CDR3 sequences of dominant TCRs. (c) An overlay of all CDR3 sequences obtained from thymocytes from indicated chimeras. CDR3 regions represented at least at 0.01% are shown. (d) The hierarchical diagrams depict similarity indices (MII) for TCR repertoires from CD4+Foxp3−and CD4+Foxp3+thymocytes (based on HTS, seeSupplementary Table1for the number of TCR CDR3 sequences analyzed). Note: the clustering of CD4+Foxp3+and CD4+Foxp3−repertoires in AbEp63KTCRmini→AbEpTCRα−chimeras was not due to their high similarity but to their low TCR diversity (seee), and the similarity between repertoires of CD4+Foxp3−subsets from AbEp63KTCRminiand AbEpKTCRmini→AbEp63KTCRα−chimeras is likely due to the negative selection by AbEp63K complex expressed on thymic medullary epithelial cells. (e) Diversity (ENS) and coverage (CVG) of TCRα CDR3 regions on CD4+Foxp3+thymocytes selected in the indicated chimeras. CD4+subsets were separately isolated from three chimeras of each kind and their TCRs were sequenced. GFP, green fluorescent protein. Figure 4: Negative selection sets apart TCR repertoires of CD4 + Foxp3 + and CD4 + Foxp3 − thymocytes. ( a ) Phenotype and recovery of thymocytes from the indicated bone marrow chimeras 6 weeks after bone marrow transplantation. Numbers indicate proportions of gated cells, and bar graphs show the mean values ±s.d. from two experiments (four mice per group). Statistical significance of data was calculated using two-sample t -test (OriginLab). ( b ) Repertoire of TCRαCDR3 regions from CD4 + Foxp3 − and CD4 + Foxp3 + thymocytes from indicated chimeras. Colour coding of the particular TCRs is the same as in Fig. 3a,b , and Supplementary Fig. 4 shows CDR3 sequences of dominant TCRs. ( c ) An overlay of all CDR3 sequences obtained from thymocytes from indicated chimeras. CDR3 regions represented at least at 0.01% are shown. ( d ) The hierarchical diagrams depict similarity indices (MII) for TCR repertoires from CD4 + Foxp3 − and CD4 + Foxp3 + thymocytes (based on HTS, see Supplementary Table1 for the number of TCR CDR3 sequences analyzed). Note: the clustering of CD4 + Foxp3 + and CD4 + Foxp3 − repertoires in A b Ep63KTCR mini →A b EpTCRα − chimeras was not due to their high similarity but to their low TCR diversity (see e ), and the similarity between repertoires of CD4 + Foxp3 − subsets from A b Ep63KTCR mini and A b EpKTCR mini →A b Ep63KTCRα − chimeras is likely due to the negative selection by A b Ep63K complex expressed on thymic medullary epithelial cells. ( e ) Diversity (ENS) and coverage (CVG) of TCRα CDR3 regions on CD4 + Foxp3 + thymocytes selected in the indicated chimeras. CD4 + subsets were separately isolated from three chimeras of each kind and their TCRs were sequenced. GFP, green fluorescent protein. Full size image Additional support for the dominant impact of negative selection on TCR repertoires of CD4 + Foxp3 + and CD4 + Foxp3 − lineages came from the analysis of CDR3 length and amino acid composition of TCRs selected on A b Ep versus A b Ep63K complexes. As shown in Fig. 5a there was a correlation between the abundance of a 10–11 amino acid-long CDR3 regions characteristic for A b Ep63K-specific TCRs and the extent of negative selection. As compared with A b wtTCR mini mice, the frequency of 10–11 amino acid-long CDR3 regions in both CD4 + subsets was strongly reduced in A b Ep63KTCR mini mice and less in A b EpTCR mini mice. Moreover, analysis of amino acid composition showed, in agreement with statistical analysis of TCR similarity, that the allocation of the same amino acid to particular position in CDR3 of the same length in both CD4 + subsets was more evident among TCRs selected on A b Ep than on A b Ep63K complexes ( Fig. 5b ). 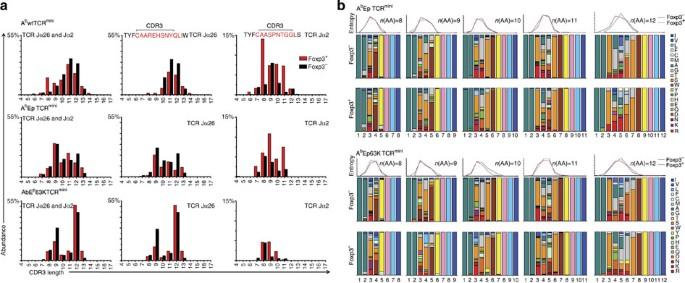Figure 5: CDR3 lengths of TCRs from CD4+Foxp3−and CD4+Foxp3+thymocytes from indicated strains. (a) Approximately 5 × 104of randomly selected CDR3 sequences from each repertoire were used for this comparison. (b) Amino acid distribution and entropy for CDR3 regions of 8–12 amino acid long from CD4+Foxp3−and CD4+Foxp3+thymocytes derived from AbEp TCRmini(upper panels) or AbEp63KTCRmini(lower panels) mice. Approximately 2 × 104of randomly selected CDR3 sequences from each repertoire were used for this comparison. This analysis was performed using IgAT software40. Figure 5: CDR3 lengths of TCRs from CD4 + Foxp3 − and CD4 + Foxp3 + thymocytes from indicated strains. ( a ) Approximately 5 × 10 4 of randomly selected CDR3 sequences from each repertoire were used for this comparison. ( b ) Amino acid distribution and entropy for CDR3 regions of 8–12 amino acid long from CD4 + Foxp3 − and CD4 + Foxp3 + thymocytes derived from A b Ep TCR mini (upper panels) or A b Ep63KTCR mini (lower panels) mice. Approximately 2 × 10 4 of randomly selected CDR3 sequences from each repertoire were used for this comparison. This analysis was performed using IgAT software [40] . Full size image TCR affinity requirements for commitment to CD4 + Foxp3 + lineage Another way to study the role of TCR in lineage commitment of CD4 + thymocytes is to analyze the frequency and distribution of TCRs that recognize selecting ligand as agonist and TCRs that do not recognize this ligand as cognate antigen. For this purpose we established a panel of A b Ep63K-specific and non-specific hybridomas from CD4 + Foxp3 + cells of Ep mice, and measured the mean fluorescence intensity of equilibrium tetramer binding to their TCRs, which provides a relative assessment of monomeric TCR:A b /peptide affinity [31] . As shown in Fig. 6a–c and Supplementary Fig. 5a , antigen responsive (#1–6) in contrast to non-responsive (#7–11) hybridomas (both responded to CD3 stimulation) stained weakly with A b Ep63K tetramer and in functional assays recognized A b Ep63 complex as an agonist ( Fig. 6b–d , Supplementary Fig. 5b ). As shown in Fig. 6e , TCRs that recognized the selecting ligand as agonist were rare or not found on CD4 + thymocytes in A b Ep63KTCR mini mice, in contrast to TCRs that did not bind this ligand with detectable affinity, which were found on both CD4 + subsets. These results also argued against the view that high affinity, self-reactive TCRs are requisite for commitment to regulatory lineage. 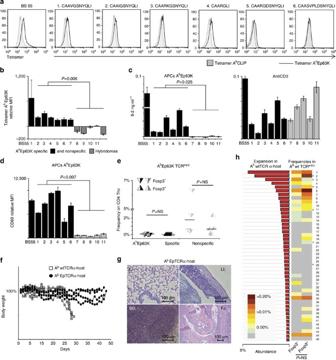Figure 6: In wild-type mice, TCR selected within the higher range of affinities are not preferentially expressed on CD4+Foxp3+thymocytes. (a) Staining of AbEp63K-specific hybridomas from AbEpTCRminimice with AbEp63K tetramer. CDR3 sequences of their TCRα chains are shown above each histogram. Staining of BS55 hybridoma served as positive and staining with AbCLIP tetramers as negative control. (b) The relative meanfluorescence index (MFI) of AbEp63K tetramer staining (±s.d. from three independent experiments) of AbEp63K-specific and non-specific hybridomas (also seeSupplementary Fig. 5a). (c) IL-2 response and (d) CD69 upregulation in response to indicated stimuli. The mean values ±s.d. from three experiments are shown (also seeSupplementary Fig.5b). (e) Frequencies of AbEp63K-specific (black/white triangles) and non-specific (grey/white triangles) TCRs on CD4+thymocytes in AbEp63KTCRminimice. Each symbol represents data from individual mice and horizontal lines show the mean value. One-way analysis of variance was used. (f) Body weight of AbwtTCRα- (squares) and AbEpTCRα- (circles) recipients of naive CD4+T cells from AbEpTCRminimice. (g) Staining by haematoxilin and eosin of tissue sections showing infiltrates of transferred AbEpTCRminiCD4+T cells in AbwtTCRα- recipients: lung (L), large intestine (LI) salivary glands (SG) and joints (FJ). (h) Frequencies of identified autoreactive TCRs in the repertoire of healthy AbwtTCRminimice (approximately one third of them were found). Heat maps represent abundance of Abwt-reactive TCRs on CD4+T cells, aligned according to their clonal expansion in response to self-peptides in lymphopenic Abwt mice. Asterisks indicate that TCR self-reactivity was confirmedin vitrousing T-cell hybridomas. Statistical significance was calculated using two-samplet-test (OriginLab). Figure 6: In wild-type mice, TCR selected within the higher range of affinities are not preferentially expressed on CD4 + Foxp3 + thymocytes. ( a ) Staining of A b Ep63K-specific hybridomas from A b EpTCR mini mice with A b Ep63K tetramer. CDR3 sequences of their TCRα chains are shown above each histogram. Staining of BS55 hybridoma served as positive and staining with A b CLIP tetramers as negative control. ( b ) The relative meanfluorescence index (MFI) of A b Ep63K tetramer staining (±s.d. from three independent experiments) of A b Ep63K-specific and non-specific hybridomas (also see Supplementary Fig. 5a ). ( c ) IL-2 response and ( d ) CD69 upregulation in response to indicated stimuli. The mean values ±s.d. from three experiments are shown (also see Supplementary Fig.5b ). ( e ) Frequencies of A b Ep63K-specific (black/white triangles) and non-specific (grey/white triangles) TCRs on CD4 + thymocytes in A b Ep63KTCR mini mice. Each symbol represents data from individual mice and horizontal lines show the mean value. One-way analysis of variance was used. ( f ) Body weight of A b wtTCRα- (squares) and A b EpTCRα- (circles) recipients of naive CD4 + T cells from A b EpTCR mini mice. ( g ) Staining by haematoxilin and eosin of tissue sections showing infiltrates of transferred A b EpTCR mini CD4 + T cells in A b wtTCRα- recipients: lung (L), large intestine (LI) salivary glands (SG) and joints (FJ). ( h ) Frequencies of identified autoreactive TCRs in the repertoire of healthy A b wtTCR mini mice (approximately one third of them were found). Heat maps represent abundance of A b wt-reactive TCRs on CD4 + T cells, aligned according to their clonal expansion in response to self-peptides in lymphopenic A b wt mice. Asterisks indicate that TCR self-reactivity was confirmed in vitro using T-cell hybridomas. Statistical significance was calculated using two-sample t -test (OriginLab). Full size image To verify our conclusions derived from analysis of ‘single-peptide’ mice we examined whether in A b wt mice, TCRs selected within the higher range of affinities are preferentially expressed on CD4 + Foxp3 + thymocytes. In healthy A b wt mice, direct identification of high affinity, self-reactive CD4 + clones is hardly possible due to their intrathymic deletion and self-tolerance. To overcome this difficulty, we first identified the TCRs specific for wt peptides in the repertoire of A b Ep63KTCR mini mice, which due to exclusive expression of single peptide are not tolerant to wt peptides. For this purpose, purified naive CD4 + T cells from A b Ep63KTCR mini mice were adoptively transferred to lymphopenic A b wtTCRα − or A b Ep63KTCRα − hosts. The former, but not the latter recipients started losing weight and developed multiorgan wasting disease ( Fig. 6f,g ), indicating that the transferred CD4 + T cells were triggered by specific, endogenous self-antigens. Then, the TCRs of in vivo expanded self-reactive CD4 + T cells were sequenced and cross-referenced to the repertoire of CD4 + thymocytes from A b wtTCR mini mice. As shown in Fig. 6h , self-reactive TCRs were randomly distributed on CD4 + Foxp3 + and CD4 + Foxp3 − thymocytes, indicating that TCRs which during positive selection bind self-peptides with high affinity are not preferentially expressed on CD4 + Foxp3 + T cells (their CDR3 lengths and sequences are shown in Supplementary Fig. 6 ). This observation supported the conclusion from the analysis of ‘single-peptide’ mice, that intrathymic commitment into CD4 + Foxp3 + and CD4 + Foxp3 − lineages is not guided by the affinity of TCR for the selecting self-peptide. Our study provides new observations of importance for understanding the intrathymic mechanisms that underlie the generation of conventional and regulatory CD4 + T cells, and mechanisms responsible for differences between their repertoires. First, CD4 + Foxp3 + thymocytes expressing diverse TCRs were efficiently generated in ‘single-peptide’ mice lacking peptide-specific niches, indicating that interactions with a restricted set of low abundant self-peptides is not obligatory for their development. Second, both subsets shared a large fraction of identical TCRs in both ‘single-peptide’ strains of mice, demonstrating that CD4 + Foxp3 + and CD4 + Foxp3 − cells can be generated from immature thymocytes as a result of recognition of the same ubiquitously expressed peptide by identical TCRs. This finding implies that TCR affinity for selecting ligand and its restricted expression in ‘thymic niches’ do not control commitment to regulatory T-cell lineage. Third, TCR repertoires of CD4 + Foxp3 + and CD4 + Foxp3 − thymocytes positively selected from CD4 + CD8 + thymocytes predominantly recognizing self-peptide with affinities from the higher end of the spectrum were less similar than the repertoires selected from CD4 + CD8 + thymocytes predominantly recognizing self-peptide with affinities from the lower end of the spectrum. This observation, together with the results from bone marrow chimeras, indicate that it is negative, not positive selection that is responsible for observed dissimilarity between the TCR repertoires of conventional and regulatory CD4 + T cells, which differ with regard to the sensitivity to apoptosis. The biological significance of this difference could stem from the fact that effectors of autoimmunity are mostly recruited from conventional T cells and therefore more stringent purging of autoreactive CD4 + Foxp3 − than CD4 + Foxp3 + thymocytes would be important for preventing ‘horror autotoxicus’. Conversely higher resistance to apoptosis of CD4 + Foxp3 + thymocytes resulting in higher TCR diversity of their positively selected progeny may be advantageous for their regulatory role in the immune system. The important question remains concerning the mechanism allowing thymocytes with the same TCR sequence to adopt different fates. As discussed in recent reviews [32] , [33] , several factors including stochastic variation in expression of molecules, can be involved and be responsible for commitment to CD4 + Foxp3 + or to CD4 + Foxp3 − lineages in normal and TCR transgenic mice; for example, predisposition of individual CD4 + CD8 + thymocytes, ‘stochastic overlap’ within intermediate range of affinities haphazardly deciding about their fate, encounter of ligand at different stages of development and/or on different antigen presenting cells, TCR-ligand dwell time and avidity. All these factors could also be involved in deciding about the fate of thymocytes with identical TCRs in single-peptide mice analyzed here, leaving open the question which of them may play the essential role. Mice The A b wtTCR mini , A b EpTCR mini , A b Ep63K strains and mice with Foxp3 GFP reporter were produced as previously described [19] , [20] , [32] . TCRα-, A b -, Ii- and A b wt mice were purchased from Jackson Laboratory. The A b wtTCR mini mice were obtained by crossing transgenic mice expressing Vα2 and Jα26 segments in germ line configuration with transgenic mice expressing TCRβ chain of the A b Ep63K-specific TCR and TCRα-mice. All mice expressing A b Ep and/or A b Ep63K complexes lacked expression of invariant chain and endogenous A b β chain, ref. 34 . To ensure that each T cell expresses only a single type of αβTCR, all TCR mini mice were heterozygous for TCR mini locus and lacked endogenous TCRα genes (TCRα−). To generate the A b Ep63KTCR mini Foxp3 GFP strain, the A b Ep63K mice were back-crossed with A b EpTCR mini Foxp3 GFP mice for eight generations. Ultimately, four new mouse strains were obtained: A b EpTCR mini Foxp3 GFP (A b EpTCR mini ), A b Ep63KTCR mini Foxp3 GFP (A b Ep63KTCR mini ) and two lymphopenic lines A b EpTCRα- and A b Ep63KTCRα-. All mice (females and males) were 6 to 8 weeks old and were housed in the laboratory animal care facility at Georgia Regents University according to the protocols approved by the Institutional Animal Care and Use Committee at our University. Phenotype analysis and cell sorting Cell surface staining with monoclonal antibodies was done by standard procedures. The following antibodies were used: anti-CD4 (clone GK1.5, 0.4 μg ml −1 ), anti-CD4 (clone RM4-5, 0.4 μg ml −1 ), anti-CD8a (clone 53–6.7, 0.4 μg ml −1 ), anti-CD25 (clone PC61, 0.4 μg ml −1 ), anti-CD5 (clone 53–7.3, 0.4 μg ml −1 ), anti-CD69 (clone H1.2F3, 0.4 μg ml −1 ), anti-TCR Vα2 (clone B20.1, 0.33 μg ml −1 ), anti-TCR Vβ14 (clone 14–2, 1.25 μg ml −1 ), anti TCRαβ (clone H57-597, 0.5 μg ml −1 ). Intra-cellular staining was performed after treatment with cell fixation/permabilization kit (eBioscience), according to the manufacturer's protocol. Antibodies used were anti-mouse Nur77 (clone 14.14, 2 μg ml −1 ) and anti-phospho-Akt (clone D9E; antibody detects endogenous levels of Akt1 only when phosphorylated at Ser473 0.5 μg ml −1 ). Monoclonal antibodies were obtained from: BD Biosciences, BioLegend or eBioscience. After staining, cells were analyzed using FACSCanto cytometer, and data were analyzed using FacsDiva software (BD Biosciences) and Flowjo V10 (TreeStar Inc.). To determine the number of the apoptotic cells within thymocytes subpopulations, after cell surface staining, the LIVE/DEAD Fixable Far-Red Dead Cell Stain Kit (Life Technologies) was used according to the manufacturer's procedure. For sorting, thymocytes or lymph node cells were stained with anti-CD4, anti-CD8 and anti-CD25 or anti-TCR Vα2. CD4 + Foxp3 + and CD4 + Foxp3 − subsets were separated on the basis of expression of Foxp3 GFP reporter. All samples were sorted using MoFlo cell sorter (Beckman Coulter) with purity>98%. Synthesis of TCR cDNA libraries and Ion Torrent sequencing Total RNA was isolated from the sorted subsets of thymocytes using RNeasey Mini Kit (Qiagen) according to the manufacturer’s procedure. Synthesis of the first complementary DNA (cDNA) strand was performed with a primer specific for the TCR Cα region (5′-TCGGCACATTGATTTGGGAGTC-3′) using Superscript III cDNA synthesis kit (Invitrogen). Incorporation of Ion Torrent sequencing primers (A-Kay and P1-Kay) to each TCR cDNA together with ‘bar-coding’ of DNA material was performed during the first amplification step using Accuprime Taq Polymerase (Invitrogen). The PCR reaction was carried out with a pair of primers specific to the Vα2 and Cα regions of the TCRα chain. The sequence of the 1st primer was as follows: 5′- CATCCCTGCGTG TCTCCGACTCAG XXXXXXXXXX GACTCTCAGCCTGGAGACT-3′, where the embolden font highlights sequence specific to the Vα2 segment of TCR, italic font marks a bar-code sequence, and the bold font is a sequence of the Ion Torrent forward sequencing primer A-Kay. The sequence of 2nd primer was as follows: 5′- CCTCTCTATGGGCAGTCGGTGATTGGT ACACAGCA GGTTCTG-3′, where embolden font highlights nucleotides specific to constant region of TCRα and bold font marks sequence of Ion Torrent reverse sequencing primer P1-Kay. After denaturation (95 °C for 2 min) four cycles of PCR proceeded as follows: three cycles at 94 °C for 15 s/54 °C for 15 s/72 °C for 40 s and one cycle 94 °C for 15 s/58 °C for 15 s/72 °C for 40 s. The obtained cDNA was cleaned using AMPure XP kit (Beckman Coulter) and used for emulsion PCR amplification according to the described protocol [35] . PCR products were cleaned again with the AMPure XP kit and the molarity of each product containing various CDR3 libraries was calculated using quantitative PCR performed with A-Kay and P1-Kay primers, according to the manufacture’s protocol (Sybergreen PCR master mix, BioRad). The libraries were mixed in equal molarity, subjected to the final amplification in the same conditions as described above, and sequenced at EdgeBio Systems (Gaithersburg, MD, USA). Low quality reads and incomplete and erroneous sequences were eliminated during data processing using filters provided by Ion Torrent Suite software. All sequences were aligned to the constant Vα2 and Cα regions and examined as described [36] . Bone marrow chimeras Sublethally irradiated, A b EpTCRα- or A b Ep63KTCRα- recipients received intravenous injection of T-cell-depleted bone marrow cells (2 × 10 6 per mouse) from A b Ep63KTCR mini or A b EpTCR mini donors, respectively. After 6 weeks CD4 + Foxp3 GFP+ and CD4 + Foxp GFP− thymocytes were sorted from each recipient and their TCRα CDR3 regions were sequenced as described above. Adoptive transfer For adoptive transfer, 2 × 10 6 of sorted CD4 + CD25 − Foxp3 GFP− cells from A b Ep63KTCR mini mice were injected intravenously to A b wtTCRα- or A b Ep63KTCRα- hosts. Mouse weight was monitored daily and the experiment was terminated when the recipient’s weight reached 80% of the starting weight. The sorted CD4 + TCRVα2 + cells from recipient’s lymph nodes and spleens were used to generate T-cell hybridomas. The antigen-specific hybridomas were identified and their TCRs were sequenced. For histology, organs were fixed with 10% neutral buffered formalin sections, cut at 8 mm, stained with haematoxylin and eosin and examined under the light microscope. T-cell hybridomas To identify Ep63K-specific TCRs, CD4 + T cells from A b EpTCR mini mice were adoptively transferred to A b Ep63KTCRα- mice, and after 8 weeks activated CD4Vα2 + T cells were sorted and expanded in vitro for 3 days in the presence of antiCD3 10 μg ml −1 and interleukin-2 (IL-2). Production of the T-cell hybridomas from CD4 + Foxp3 − and CD4 + Foxp3 + cells and an in vitro IL-2 assay were previously described [14] , [37] . Reponses of hybridomas to antigen presenting cells presenting Ep63K complexes were determined based on change in the relative expression of CD5 and CD69 using standard flow cytometry procedures, and by detecting the amount of IL-2 produced following activation [14] . The two-sample t -test and one-way analysis of variance test was used to calculate statistical significance. Tetramer staining To stain hybridomas with A b Ep63K and A b CLIP tetramers, 5 × 10 4 cells were incubated with anti-CD4 (clone GK1.5) 0.4 μg ml −1 and anti-TCR (clone H57-597) 0.5 μg ml −1 antibodies, respectively, to crosslink TCRs, then gently washed and incubated additionally for 4 h with A b Ep63K 10 μg ml −1 or A b CLIP 10 μg ml −1 (control) tetramers. The optimal concentrations of tetramers used for staining were estimated experimentally. Both tetramers were synthesized by NIH-supported Tetramer Core at Emory University (Atlanta, GA, USA). Binding of A b Ep63K and A b CLIP tetramers to the TCR-expressing hybridomas was then analyzed by flow cytometry. Statistical methods Statistical analysis was performed using the R statistical software (R 2.15.0). For the comparative analysis of the overlap, a mutual information index (I-index) was used as defined [28] together with a hierarchical (agglomerative) clustering procedure with Ward linkage method [38] . Stability of clustering was assessed via parametric (multinomial) bootstrap—the 95% confidence bounds for similarity matrices were constructed based on the Frobenius norm. The sample coverage (CVG)—that is, the conditional probability of discovering a new receptor—was estimated according to the Good–Turing formula [39] . The CVG index was calculated using a resampling procedure (multinomial bootstrap) with varying sample sizes (from fifty up to the size of the original sample) to assess the effect of under-sampling on the analysis. Diversity was quantified using the effective number of species and presented in the form of diversity profiles (for definitions see ref. 28 ). These profiles are plots of the order of the index versus the value of the index, thus enabling comparisons of diversity with more weight put on rare (the order of index lower than one) or abundant (the order of index higher than one) receptors. The 95% confidence bounds were constructed as described above. The significance of differences between individual samples or groups of mice was determined by two-sample t- test and one-way analysis of variance test using Origin 9.1 software, and P -values<0.05 were considered statistically significant. How to cite this article: Wojciech, L. et al. The same self-peptide selects conventional and regulatory CD4 + T cells with identical antigen receptors. Nat. Commun. 5:5061 doi: 10.1038/ncomms6061 (2014).